Biological carbon precursor to diagenetic siderite with spherical structures in iron formations During deposition of Precambrian iron formation, the combined sedimentation of ferrihydrite and phytoplankton biomass should have facilitated Fe(III) reduction during diagenesis. However, the only evidence for this reaction in iron formations is the iron and carbon isotope values preserved in the authigenic ferrous iron-containing minerals. Here we show experimentally that spheroidal siderite, which is preserved in many iron formation and could have been precursor to rhombohedral or massive siderite, forms by reacting ferrihydrite with glucose (a proxy for microbial biomass) at pressure and temperature conditions typical of diagenesis (170 °C and 1.2 kbar). Depending on the abundance of siderite, we found that it is also possible to draw conclusions about the Fe(III):C ratio of the initial ferrihydrite-biomass sediment. Our results suggest that spherical to rhombohedral siderite structures in deep-water, Fe-oxide iron formation can be used as a biosignature for photoferrotrophy, whereas massive siderite reflects high cyanobacterial biomass loading in highly productive shallow-waters. Iron formations (IFs) are marine chemical sedimentary rocks that were precipitated throughout much of the Archaean and Paleoproterozoic before ~1.85 Ga ( [1] ). The precursor sediments, including amorphous ferric oxyhydroxides, such as ferrihydrite (Fe(OH) 3 ), required an oxidative mechanism to transform the dissolved hydrothermally-derived Fe(II) into solid-phase Fe(III). It has been suggested that abiotic UV-light dependent oxidation of Fe(II) led to the precipitation of ferric hydroxide minerals [2] , [3] , but later experiments have shown that in seawater containing high concentrations of dissolved Si(OH) 4 and HCO 3 − the oxidation effects of either UVA or UVC are negligible compared to the precipitation of ferrous iron-silicates [4] . In contrast, two different roles for bacteria have been inferred in Fe(II) oxidation. The first is based on the production of O 2 by oxygenic phototrophic cyanobacteria. Their Precambrian ancestors flourished when nutrients were available and their metabolically-produced O 2 abiotically oxidized dissolved Fe(II) to Fe(III), followed by the hydrolysis and precipitation of ferrihydrite [5] . The second postulated role for bacteria in IF precipitation involves Fe(II)-oxidizing microorganisms, including microaerophilic chemolithoautotrophic bacteria (for example, Gallionella ferruginea ) that thrive today in suboxic waters and sediments [6] . Additionally, anoxygenic photoautotrophic Fe(II)-oxidizing bacteria (photoferrotrophs) may have coupled the C and Fe cycles before the evolution of oxygenic photosynthesis [7] , [8] , [9] . A number of experimental studies have confirmed that various purple and green phototrophic bacteria can use Fe(II) as a reductant for CO 2 fixation [10] . However, the relative influence of phototrophic bacteria on the origin of IF is not fully understood, because direct evidence for their involvement in Fe(II) oxidation has not been found and the fate of organic remains and ferrihydrite precipitates on the seafloor are still poorly characterized. Given that the bulk of the ocean water column was anoxic throughout the Archaean and Paleoproterozoic, ferrihydrite represented a favourable electron acceptor for in situ oxidation of the cellular biomass remains associated with precursor IF sediments. Some Archaean magnetite-rich IF [11] , [12] , [13] , [14] , [15] have highly negative δ 56 Fe values that are comparable to those measured from dissolved Fe(II) experimentally produced by cultures of dissimilatory Fe(III)-reducing bacteria [16] , pointing to the antiquity of anaerobic dissimilatory Fe(III) reduction [15] , [17] . Alternatively, abiotic reactions between Fe(III) oxyhydroxides and organic carbon are expected to occur at temperatures above the threshold for microbial life during late-stage diagenesis and metamorphism [18] , which based on modern microbes is around 120 ° C ( [19] ). In either case, coupling the reduction of Fe(III) minerals to the oxidation of organic matter provides a simple explanation for the generally low content of organic carbon in IF (<0.5% ( [1] , [20] )), as well as the light carbon and iron isotopic values of carbonate minerals [1] , [15] , [21] , [22] . A number of petrographic studies have described the secondary origin of magnetite in IF [23] , [24] , [25] , [26] . Recently, Li et al . [27] reported the detection of nanocrystals of apatite in association with magnetite from the 2.48 Ga Dales Gorge IF in Western Australia; the latter had a crystal chemistry identical to modern biogenic magnetite. These considerations and features point to the original presence of biomass in IF precursor sediments, but also indicate that the organic carbon served as an electron donor during Fe(III) reduction. Beside magnetite and haematite, siderite is one of the most abundant Fe-bearing minerals in IF. The origin of siderite has been suggested to involve primary precipitation in the water column through the reaction of Fe 2+ with bicarbonate from seawater as soon as the solubility product of siderite (controlled by the Fe 2+ and carbonate/bicarbonate concentrations in the ocean water) is exceeded [28] , [29] . Alternatively, siderite can be formed during the diagenetic (biological or non-biological), and subsequent metamorphic, oxidation of microbial biomass to CO 2 /bicarbonate coupled to the reduction of Fe(III), followed by reactions of the product Fe 2+ with the sediment pore-water bicarbonate [30] . Here, we show that spherical siderite in deep-water IF represents a biosignature for photoferrotrophy, whereas massive siderite reflects high cyanobacterial biomass in shallow-water. Experimental siderite formation We experimentally tested whether the diagenetic transformation of biomass and primary Fe(III) oxyhydroxide minerals can form siderite, and whether that siderite is of similar size and morphology to those observed in IF. To this end, we incubated ferrihydrite (as a proxy for primary ferric oxyhydroxides) and glucose (as a proxy for microbial biomass) in gold capsules at 170 °C and 1.2 kbar (for a more detailed rationale explaining the choice of reactants and for methodological details see Supplementary Information ). These chosen conditions simulate the degree of metamorphism in some of the major IF in South Africa and Western Australia that have been exposed to metamorphic grades below the prehnite-pumpellyite facies [31] , [32] , [33] . After 24 h of incubation, haematite, magnetite and siderite were identified as reaction products by their optical properties ( Fig. 1 ). Detailed microscopic analysis showed that the siderite was commonly present as spherical grains characterized by strong bireflectance and anisotropism ( Fig. 2a ). As no significant concentrations of Mg 2+ and Ca 2+ were present in our experiments, we deduce that the carbonate spheres are siderite. This has also been independently confirmed by Mössbauer spectroscopy and XRD (data not shown). 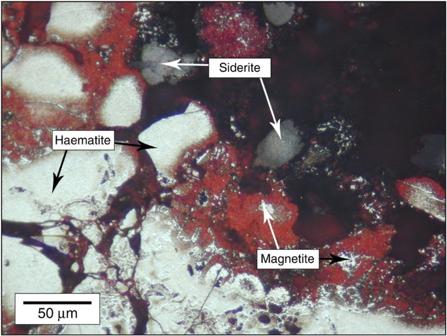Figure 1: Iron(II) and iron(III) minerals formed during pressure-temperature diagenesis. Reflected light microscopy image of a mixture of ferrihydrite and glucose after 1 day of pressure and temperature treatment at 1.2 kbar and 170 °C, respectively. Haematite and magnetite have formed along with siderite. All three minerals can be found in close association with each other. Haematite forms large anhedral to subhedral crystals, which show small magnetite inclusions. Siderite is present as the typical grey sub-spherical structures. Figure 1: Iron(II) and iron(III) minerals formed during pressure-temperature diagenesis. Reflected light microscopy image of a mixture of ferrihydrite and glucose after 1 day of pressure and temperature treatment at 1.2 kbar and 170 °C, respectively. Haematite and magnetite have formed along with siderite. All three minerals can be found in close association with each other. Haematite forms large anhedral to subhedral crystals, which show small magnetite inclusions. Siderite is present as the typical grey sub-spherical structures. 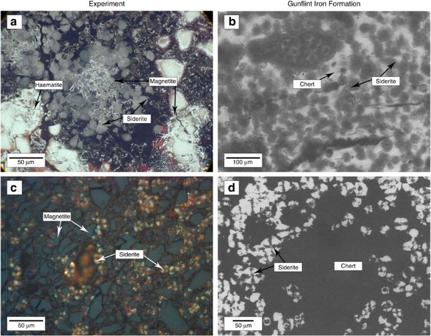Figure 2: Spherical siderite structures in diagenesis experiments and Precambrian IFs. Reflected light microscopy images of siderite spheres formed in diagenetic experiments from a mixture of ferrihydrite and glucose (a,c) compared with spherical siderite structures in IF (b,d). Ferrihydrite and glucose with an electron ratio of 0.6 was treated at 1.2 kbar and 170 °C for 14 days. (a) Shows haematite, magnetite and spherical siderite formed in the diagenetic experiments in comparison to analogous spherical siderite structures in chert from the Gunflint IF near Kakabeka Falls, Ontario (b). (c) Ferrihydrite and glucose mixture (electron ratio of 2.4) under crossed polars. Magnetite is surrounded by siderite spheres that show distinct polarization crosses. These spheres are similar to siderite structures in the carbonate facies of the upper and lower Gunflint IF, Ontario34. Full size image Figure 2: Spherical siderite structures in diagenesis experiments and Precambrian IFs. Reflected light microscopy images of siderite spheres formed in diagenetic experiments from a mixture of ferrihydrite and glucose ( a , c ) compared with spherical siderite structures in IF ( b , d ). Ferrihydrite and glucose with an electron ratio of 0.6 was treated at 1.2 kbar and 170 °C for 14 days. ( a ) Shows haematite, magnetite and spherical siderite formed in the diagenetic experiments in comparison to analogous spherical siderite structures in chert from the Gunflint IF near Kakabeka Falls, Ontario ( b ). ( c ) Ferrihydrite and glucose mixture (electron ratio of 2.4) under crossed polars. Magnetite is surrounded by siderite spheres that show distinct polarization crosses. These spheres are similar to siderite structures in the carbonate facies of the upper and lower Gunflint IF, Ontario [34] . Full size image Siderite was present in close association with ferrihydrite and haematite, suggesting that the reduction of ferrihydrite or haematite coupled to the oxidation of biomass (for example, glucose) formed siderite, Fe 2+ , OH − , and potentially even H 2 , according to the following four reactions: 4Fe(OH) 3 +CH 2 O→FeCO 3 +3Fe 2+ +6OH − +4H 2 O 2Fe 2 O 3 +CH 2 O+2H 2 O→FeCO 3 +3Fe 2+ +6OH − 2Fe(OH) 3 +2CH 2 O→2FeCO 3 +2H 2 O+3H 2 Fe 2 O 3 +2CH 2 O+H 2 O→2FeCO 3 +3H 2 Comparison with siderite in IFs Our experiments show that spherical siderite can form from the abiotic diagenetic oxidation of organic carbon coupled to a reduction of ferric iron during simulated late-stage diagenesis ( Fig. 2a ). Figure 2b show a comparison of diagenetically formed siderite spheres in our experiments with spherical siderite structures in the 1.88 Ga Gunflint IF in Canada [34] , [35] , [36] , [37] , [38] . Siderite spheres with sizes of tens of microns can be observed in both the experimental and natural mineral assemblages where they appear as individual grains as well as in the form of aggregates when the grains coalesce. Similar structures of spherical siderite have also been described in IFs in the 2.48 Ga Dales Gorge Member, Western Australia [39] , [40] and 1.88 Ga Riverton IF, Michigan, MI, USA [41] , although they are not as common in these successions as in the Gunflint IF. Such occurrences suggest that siderite spheres may have been a common feature of IFs before they were recrystallized during late diagenesis and metamorphism to rhombohedral/subhedral siderite grains or formed massive siderite beds. Consistent with this suggestion, it has been shown that in the Gunflint IF some siderite rhombohedra contain spheres in their cores and there is a clear progression from siderite spheres to siderite rhombohedra without any trace of spheres left [37] , [42] . This progression was also found in the Dales Gorge Member, where siderite spheres and rhombohedra occur in close proximity to each other ( Fig. 3c ). Note that some spheres already show signs of a recrystallization. 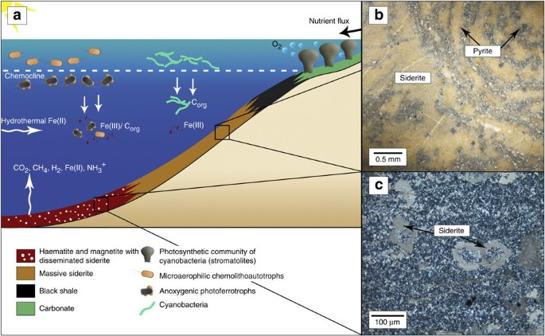Figure 3: Origin of massive siderite beds and spherical siderite structures in different depositional environments. Model summarizing the origin of shallow- and deep-water IF siderite (a). During periods of enhanced submarine volcanism, hydrothermal fluids leached Fe(II) from volcanics and exhaled it to the oceans. Fe(II) upwelling from the deep ocean resulted in the growth of microaerophilic chemolithoautotrophs and anoxygenic photoferrotrophs in the deep-water, photic zone above and below the chemocline, respectively. Due to low-cell densities in the active Fe(II)-oxidation zone and a much smaller Corgreduction potential in sediments with respect to the accumulated Fe(III), haematite and magnetite with disseminated spherical to rhombohedral siderite formed during diagenesis. By contrast, high riverine nutrient fluxes to shallow-water environments led to cyanobacterial blooms; this resulted in a C:Fe ratio of 1:4 or more, which is equal to or greater than the reduction ratio in sediments. This led to the formation of large quantities of siderite grains, which coalesced during diagenesis and metamorphism to form massive siderite beds. (b) Massive siderite beds formed in a shallow-water environment in association with stromatolites (with lamina highlighted by pyrite crystals) in the volcanically-dominated ca. 2.7 Ga Michipicoten greenstone belt, Wawa subprovince of the Superior province, Canada (reflected light image, Helen IF, MacLeod mine51). (c) In the deeper-water environments, sub-spherical to rhombohedral siderite structures formed during early diagenesis to low-grade metamorphism of IFs as shown in the photomicrograph under cross-nicols of the ca. 2.48 Ga Dales Gorge IF of Western Australia. Figure 3: Origin of massive siderite beds and spherical siderite structures in different depositional environments. Model summarizing the origin of shallow- and deep-water IF siderite ( a ). During periods of enhanced submarine volcanism, hydrothermal fluids leached Fe(II) from volcanics and exhaled it to the oceans. Fe(II) upwelling from the deep ocean resulted in the growth of microaerophilic chemolithoautotrophs and anoxygenic photoferrotrophs in the deep-water, photic zone above and below the chemocline, respectively. Due to low-cell densities in the active Fe(II)-oxidation zone and a much smaller C org reduction potential in sediments with respect to the accumulated Fe(III), haematite and magnetite with disseminated spherical to rhombohedral siderite formed during diagenesis. By contrast, high riverine nutrient fluxes to shallow-water environments led to cyanobacterial blooms; this resulted in a C:Fe ratio of 1:4 or more, which is equal to or greater than the reduction ratio in sediments. This led to the formation of large quantities of siderite grains, which coalesced during diagenesis and metamorphism to form massive siderite beds. ( b ) Massive siderite beds formed in a shallow-water environment in association with stromatolites (with lamina highlighted by pyrite crystals) in the volcanically-dominated ca. 2.7 Ga Michipicoten greenstone belt, Wawa subprovince of the Superior province, Canada (reflected light image, Helen IF, MacLeod mine [51] ). ( c ) In the deeper-water environments, sub-spherical to rhombohedral siderite structures formed during early diagenesis to low-grade metamorphism of IFs as shown in the photomicrograph under cross-nicols of the ca. 2.48 Ga Dales Gorge IF of Western Australia. Full size image Influence of initial Fe(III):C ratios on siderite formation In order to determine how varying levels of biomass might influence siderite formation and the internal morphology of spheres, we performed a second series of experiments using four times more glucose. The electron ratio, calculated with the total number of electrons potentially released from carbon in glucose divided by the number of electrons that can potentially be accepted by the Fe(III), was thus increased from 0.6 in the first experiments to 2.4 (see Supplementary Information ). Experiments with an electron ratio of 0.6 simulate an excess of iron as would have occurred in a scenario in which the Fe 2+ would be oxidized by anoxygenic photoferrotrophs (for example, Chlorobium sp.) or microaerophilic chemolithoautotrophs (for example, Gallionella sp.) ( Fig. 3 ): preferential deposition of the dense Fe(III) minerals with low content of organic carbon has been demonstrated experimentally for photoferrotrophs [43] . In comparison, an electron ratio of 2.4 represents a system with a higher biomass input to the sediment as would be the case if there was either additional electron donors such as H 2 , or if a microbial metabolism, such as photosynthesis by cyanobacteria, occurred in the water column and was not directly tied to Fe(II) oxidation. Our diagenesis experiments showed that siderite formed at both electron ratios and that it most commonly had a spherical shape (shown by black and white arrows in Fig. 2a ) up to 20 μm in diameter. Individual spheres sometimes coalesced to form aggregates. Associated with the siderite were haematite (in experiments with an electron ratio of 0.6) and magnetite (in both experiments). Magnetite was commonly found to be interspersed with haematite grains or as rims around haematite cores. In the experiment with an electron ratio of 2.4, magnetite grains were larger and often surrounded by siderite ( Fig. 2c ). The sub-spherical siderite crystals in the 2.4 electron ratio experiments showed distinct polarization crosses under crossed polars ( Fig. 2c ), suggesting either concentrical or radial crystal growth in siderite spheres [34] , [44] . Polarization crosses under crossed polars and radial crystal growth were only observed in capsules with a higher electron ratio, but were also observed in siderite spheres from the Gunflint IF ( Fig. 2d ; see also ref. 45 ) and from the Riverton IF of the Iron River district, Michigan [41] . The results thus suggest that these structures can be considered as an indicator for high organic carbon loading into the sediments. Consistent with this suggestion, siderite spheres in IFs often contain organic carbon inclusions [42] . To our knowledge, polarization crosses under crossed polars have not yet been described for siderite minerals formed by microbial reduction of Fe(III) minerals either in laboratory or in nature. Therefore, by comparison with previously described siderite spheres in IF, our experiments suggest that at least some siderite spheres were formed by abiotic diagenetic formation of siderite via reduction of Fe(III) oxyhydroxides with biomass. Influence of silica on siderite formation To test whether spherical siderite would also form in the presence of Si concentrations similar to those expected for the Archaean oceans, we carried out experiments with Si-coated ferrihydrite and glucose (Si:Fe ratio of 0.08, electron ratio 0.6, for details see Supplementary Information ). We found that in the presence of Si, siderite also formed within 14 days and was visible both as individual spheres and as aggregates ( Fig. 4 ). 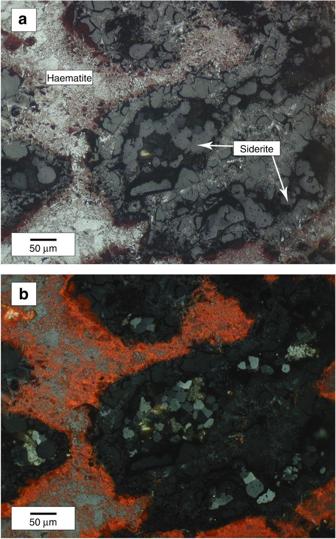Figure 4: Iron(II) and iron(III) minerals formed during pressure-temperature diagenesis in the presence of silica. Reflected light microscopy image (a) of minerals formed in diagenetic experiments with a mixture of silica-coated ferrihydrite and glucose (Si:Fe ratio of 0.08, electron ratio 0.6). Siderite is visible as aggregates and as single globular structures.bshows an image of the same area under crossed polars. Figure 4: Iron(II) and iron(III) minerals formed during pressure-temperature diagenesis in the presence of silica. Reflected light microscopy image ( a ) of minerals formed in diagenetic experiments with a mixture of silica-coated ferrihydrite and glucose (Si:Fe ratio of 0.08, electron ratio 0.6). Siderite is visible as aggregates and as single globular structures. b shows an image of the same area under crossed polars. Full size image Although siderite can form via both abiotic and biotic mechanisms [21] , [17] , [30] , specific petrographic features of spherical siderite in IF have been suggested to represent remnants of microbial cells based on their shape and internal structure [35] , [36] . Heaney and Veblen [34] argued for an indirect biological origin of nano-scale siderite spheres from the Gunflint IF as distinct cores of apatite were found within the siderite spheres. Based on a simple mass-balance analysis, they inferred that it was the accumulation of ‘thousands of individual organisms’ that accounted for the relatively high amount of apatite inside of the spheres and for the spheres themselves. However, the described structures in the Gunflint IF have a size range between 24–115 μm (Kazmierczak et al . [35] and Fig. 2b ), and thus do not resemble the typical size of bacterial cells. In either case, several IF, including the Dales Gorge Member of Western Australia [39] , [40] , the Riverton IF in Michigan [41] , and the Gunflint IF in Ontario [38] , have been reported to contain these distinctive structures. The presence of spherical siderite in IFs with different ages and from varied depositional settings, shallow and deep marine, suggests a common mechanism of their formation. A key conclusion from our experiments is that the presence of siderite in IFs may allow a first-order estimate of the initial amount of sedimentary organic matter, and potentially even characterization of the ecosystem that grew in the photic zone during IF deposition. Using the Dales Gorge Member as an example, we calculated that based on measured Fe TOTAL content, a plausible depositional rate of 1 mm per year [46] , and a post-precipitation reduction efficiency of 70% before burial [47] , the amount of Fe(III) precipitated could have been as high as 45.3 mol per year × m 2 (for details of calculation see Supplementary Information ). Using an experimental rate of Fe(II) oxidation of 1.1 × 10 −11 mol per cell by chemolithoautotrophic bacteria [48] , such as Gallionella ferruginea (one of the species believed to have played a prominent role in ferric iron precipitation in some IF [49] —see SOM), it is further possible to estimate the cell density of bacteria growing in the photic zone of early Precambrian seawater, as the rate of Fe(III) precipitation estimated above would necessitate population of chemolithotrophic bacteria on the order of 10 5 cells per ml (for details of calculation see Supplementary Information ) throughout the Fe(II) oxidation zone of the water column with a biologically active depth of 10 m. Similar cell density would have existed if Fe(II) oxidation was primarily driven by photoferrotrophic bacteria. Putting these numbers into context, we can envision two different scenarios that would have ultimately led to the different diagenetic/metamorphic minerals found in IF ( Fig. 3 ). It has long been recognized that in Neoarchean-early Paleoproterozoic IF-bearing basins with a well-preserved shallow- to deep-water depositional profile, deep-water Fe-oxide facies grade into shallow-water Fe-carbonate facies [28] . We suggest that during periods of high Fe(II) upwelling, the deep-water, photic zone (that also contained low O 2 concentrations due to the activity of cyanobacteria) was populated with Gallionella -type cells above the chemocline and Chlorobium -type cells below the chemocline, but throughout the active Fe(II) oxidation zone, cell densities were on average 10 5 cells per ml or less. As Gallionella , in particular, forms Fe(III) with a C:Fe ratio of 1:6, but the reduction of Fe(III) in sediments with dead biomass has a C:Fe ratio 1:4, then excess Fe(III) is accumulated, leading to haematite and magnetite formation with small amount of disseminated siderite found in most deep-water IF, such as the Dales Gorge Member ( Fig. 3 ). This also applies for photoferrotrophic bacteria, as shown by Posth et al . [43] , due to only partial deposition of the biomass while all precipitated Fe(III) minerals sediment to the ocean floor. By contrast, in the shallow-water environments, where only a limited amount of upwelling Fe(II) was supplied, the relative numbers of photoferrotrophs/ Gallionella were lower (because their electron donor Fe 2+ is limiting under such conditions), whereas higher riverine nutrient input could have resulted in cyanobacterial blooms. This would have led to the production of ferric iron (via the indirect reaction of O 2 with ferrous iron) at a C:Fe ratio of 1:4 (or even greater). This is equivalent to, or even greater, than the reduction ratio, thereby minimizing the amount of Fe(III) buried. Importantly, the cyanobacteria would have produced biomass that was not tied to Fe(II) oxidation, thereby increasing the overall C:Fe ratio in the sediments. Furthermore, given the possibility that significant concentrations of H 2 were also present (via fermentation) in the water column [50] , autotrophic photosynthesis decoupled from Fe(II) oxidation would have also added biomass, causing a rise in the C:Fe ratio. Therefore, massive siderite with precursor spherical siderite would have formed in the transition zone to the shallow-water environments. Such siderites have been described in the ca. 2.7 Ga Helen iron formation, Ontario [51] . Disseminated siderite spheres or, at higher metamorphic grade, rhombohedral to anhedral-subhedral siderite grains, however, would be preserved in deep-water, Archaean Fe-oxide facies IF ( Fig. 3c ). Consistent with this ecological zonation, stromatolites have been described from massive siderite deposits [51] ( Fig. 3b ), whereas disseminated siderite spheres and, more commonly, rhombohedral to anhedral-subhedral siderite grains were found in the Gunflint [34] , [35] , [36] , [37] , [38] , Riverton [41] and Dales Gorge Fe-oxide facies IF [39] , [40] . Although a biological role for the origin of IF has been suggested in the past [24] , we have, for the first time, provided experimental evidence that organic biomass in association with Fe(III) mineral precipitates forms spherical siderite structures under diagenetic conditions. This, in turn, can be used to argue for the presence of cellular biomass in association with the primary Fe(III) precipitates in IF, thereby implying that biological activity was indeed involved in IF deposition. Perhaps most intriguingly, the abundance of siderite in IF might also be used to estimate the initial amount of sedimentary organic matter in Precambrian ferruginous marine environments and its predominant style of metabolism. Our study points to diverse microbial communities in the Archaean oceans with the shallow-water environments populated by cyanobacterial communities, whereas photoferrotrophs and microaerophilic chemolithoautotrophs were abundant in the deep-water photic zone. Setup and analysis of gold capsule diagenesis simulation experiments Ferrihydrite (chemically synthesized) and glucose (as proxy for biogenic Fe(III) precipitates and microbial biomass) were weighted, mixed and carefully homogenized before they were filled into 3 cm long gold capsules, which were cut from a 1-m long gold tube with an outer diameter of 2.5 mm and a wall thickness of 0.2 mm. The capsules were filled with 100 mg of ferrihydrite and with either 4.23 or 16.9 mg glucose. The lower amount of glucose represents an electron ratio of 0.6, which is the ratio of the electrons potentially released from the carbon in the glucose divided by the electrons potentially accepted by the Fe(III) in the ferrihydrite. The larger amount of glucose represents an electron ratio of 2.4. After the filling, the capsules were closed mechanically and sealed with an arc welding. Closed capsules were then placed into rapid quench autoclaves for pressure and temperature treatment at 1.2 kbar and 170 °C for 14 days. To stop the reactions, capsules were dropped from the sample chamber into the water-cooled part of the autoclave. After incubation, the capsules were either prepared as thick sections and embedded in epoxy resin for identification of the mineral phase content and the mineral spatial arrangement by reflected light microscopy, or the material inside the capsules was taken out for Mössbauer spectroscopy and XRD to identify the iron mineral phases. How to cite this article: Köhler, I. et al . Biological carbon precursor to diagenetic siderite with spherical structures in iron formations. Nat. Commun. 4:1741 doi: 10.1038/ncomms2770 (2013).